Resolving cancer–stroma interfacial signalling and interventions with micropatterned tumour–stromal assays Tumour–stromal interactions are a determining factor in cancer progression. In vivo, the interaction interface is associated with spatially resolved distributions of cancer and stromal phenotypes. Here, we establish a micropatterned tumour–stromal assay (μTSA) with laser capture microdissection to control the location of co-cultured cells and analyse bulk and interfacial tumour–stromal signalling in driving cancer progression. μTSA reveals a spatial distribution of phenotypes in concordance with human oestrogen receptor-positive (ER+) breast cancer samples, and heterogeneous drug activity relative to the tumour–stroma interface. Specifically, an unknown mechanism of reversine is shown in targeting tumour–stromal interfacial interactions using ER+ MCF-7 breast cancer and bone marrow-derived stromal cells. Reversine suppresses MCF-7 tumour growth and bone metastasis in vivo by reducing tumour stromalization including collagen deposition and recruitment of activated stromal cells. This study advocates μTSA as a platform for studying tumour microenvironmental interactions and cancer field effects with applications in drug discovery and development. Epithelial cancer progression is associated with an evolving tissue interface of direct epithelial–stromal interactions [1] . In human tumour biopsies, extensive gene expression changes are correlated with cancer staging on both sides of the tumour–stroma interface [2] , [3] ; importantly, some epithelial–mesenchymal transition (EMT) signatures are preferentially expressed by cancer cells close to the interface, while interfacial stromal fibroblasts promote EMT more effectively than those extracted from the bulk millimetres away [4] , [5] . It is, however, extremely difficult to clarify the exact, cell-specific contribution of tumour–stromal interactions in the development of this structure–function relationship in cancer progression in vivo because of a lack of experimental control [6] . Conventional in vitro models use random or transwell co-cultures to study contact- or soluble factor-mediated tumour–stromal signalling and screen for new drugs [7] , [8] . However, in real tumours, cells at the tissue bulk and interface can be simultaneously and differentially influenced by the extent of heterotypic cell–cell contact and the long/short-range diffusion of soluble factors [9] . These models that indiscriminately mix two or more cell types cannot resolve this critical spatial perspective of tumour–stromal interactions, nor accurately assess drug action mechanisms in the heterogeneous cell compartments in the bulk and at the interface. Micro-engineered cell cultures have emerged as powerful platforms to model processes in tissue microenvironments at appropriate length scales and identify their impact on cell morphogenesis and differentiation [10] , [11] , [12] , [13] . Yet, the downstream analysis of micro-engineered cultures (as well as conventional cultures) has largely relied on resource-demanding immunocytochemistry, or mechanochemical cell isolation to understand cell-specific phenomena, which introduces additional experimental artifacts and results in a loss of information on the original location of cells. Microscopy-based laser capture has been used to retrieve cells in micropatterns for gene expression analysis [14] . However, the spatial resolution of the technique was not fully leveraged, and its combined use with micro-engineered cell co-cultures to understand spatially-defined signalling in cancer progression and drug actions has not been demonstrated to date. A micropatterned tumour–stromal assay (μTSA) is established to organize tumour and stromal cells into distinct, spatial compartments with a defined heterotypic cell interface. By integrating μTSA with microscopy and laser capture microdissection (LCM), we enable cell-specific analysis of phenotypes and gene expression in situ with precise spatial resolution. Using μTSA, we reveal a preferential instigation of malignant tumour–stromal signalling by bone marrow fibroblasts. Tumour cell expression profiles in μTSA are benchmarked against human ER+ breast cancer tissue and found to have 63% concordance using a defined set of genes related to cancer progression. The co-culture system is further adapted to evaluate a new mechanism of action by known cancer therapeutics to disrupt tumour–stromal interfacial interactions with prediction of μTSA observations in vivo . Below, we present μTSA as a tool to explore a new frontier of tumour–stromal interfacial interactions with the underlying hypothesis that bulk and interfacial tumour cells can be differentially influenced by the type of neighbouring stromal cell or a pharmacological intervention. Micropatterning to control a tumour–stroma interface Micropatterned tumour–stromal assays (μTSAs) were designed to organize tumour and stromal cells into distinct, spatial compartments in vitro with a defined heterotypic cell interface by a stencil micropatterning technique [12] , [15] ( Fig. 1a ), mimicking in vivo constraints on contact- and paracrine-signalling in the context of a growing tumour–stroma boundary layer. A cell-repellent, silicone mask was created with circular apertures that were cut by laser to form a cell culture stencil. The stencil mask defined the shape and size of areas where cancer cells initially attached and formed small multicellular islands ( Fig. 1a ). Stromal cells were seeded to occupy the rest of the area after removal of the stencil, thereby creating a pre-determined tumour–stromal interaction interface (see Methods). Breast cancer and fibroblastic stromal cells were selected on the basis of known stroma-induced tumour activity [16] . 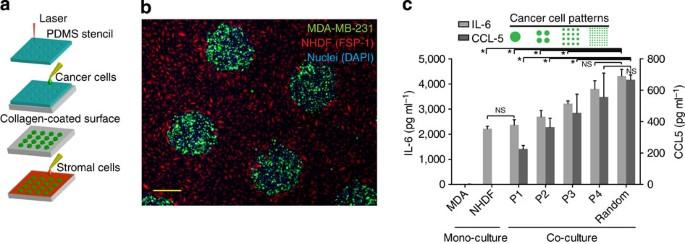Figure 1: Heterotypic cell–cell interactions are precisely controlled in micropatterned tumour–stromal assay (μTSA). (a) Schematics of the μTSA fabrication process. (b) μTSA co-culture of MDA-MB-231 (expressing GFP) breast cancer cell with normal human dermal fibroblasts (NHDF) (stained for fibroblast-specific protein-1, FSP-1). Scale bar, 100 μm. (c) Forty-eight-hour IL-6 and CCL5 secretion in MDA and NHDF mono-cultures, random and μTSA co-cultures with four different micropattern designs. NS, not significant; *P<0.05, by one-way analysis of variance. (c)n=3. Error bars: s.d. Figure 1b shows a μTSA of breast cancer cell MDA-MB-231 (engineered to express GFP [17] ) and normal human dermal fibroblast (NHDF; stained for FSP-1) 24 h after initial seeding. Notably, μTSA allows for seeding a fixed number of cancer and stromal cells while varying the total length of tumour–stromal interfaces ( Supplementary Fig. 1 ). To demonstrate that an increased tumour–stromal interface would correlate with cancer-induced stromal function, MDA-MB-231 and NHDF were cultured in four representative seeding patterns in μTSA ( Fig. 1c inset). Stromal secretion of IL-6 (ref. 18 ) and CCL5 (ref. 17 ), two tumour-inducing factors, increased as a function of tumour–stromal interfaces between MDA and NHDF cells, with a maximal found in random co-culture ( Fig. 1c ). The data suggest that the activation/sensitization of stroma by tumour cells is exquisitely controlled by direct contact. Figure 1: Heterotypic cell–cell interactions are precisely controlled in micropatterned tumour–stromal assay (μTSA). ( a ) Schematics of the μTSA fabrication process. ( b ) μTSA co-culture of MDA-MB-231 (expressing GFP) breast cancer cell with normal human dermal fibroblasts (NHDF) (stained for fibroblast-specific protein-1, FSP-1). Scale bar, 100 μm. ( c ) Forty-eight-hour IL-6 and CCL5 secretion in MDA and NHDF mono-cultures, random and μTSA co-cultures with four different micropattern designs. NS, not significant; * P <0.05, by one-way analysis of variance. ( c ) n =3. Error bars: s.d. Full size image Ki-67 evolves within μTSA under an inhibitory environment NHDFs were previously reported to inhibit tumour cell proliferation [19] . μTSA was used to evaluate this purported anti-proliferative activity at the interface. Ki-67 in μTSA was measured as a proliferation marker in MDA-MB-231 cultures with or without NHDFs. Ki-67 remained predominantly expressed in MDA-MB-231 cells over time ( Fig. 2a ). Ki-67 intensity of individual cells was plotted against their radially normalized location in the micropattern ( Fig. 2b,c ). MDA-MB-231 cells had significantly higher Ki-67 in monoculture (Student’s t -test, P <0.01) than in co-culture with NHDF ( Fig. 2d ). Interestingly, we saw an initial decrease in Ki-67 expression at day 2 in both conditions, followed by increased expression afterwards, suggesting a synchronization of cancer cell cycles when cultured in a micropatterned format ( Fig. 2d ). Ki-67 density in MDA-MB-231 monoculture patterns showed a distinct spatial abundance in the periphery over time. In co-culture with NHDF, Ki-67 expression was static and revealed a spatial impact of NHDF on the distribution of MDA-MB-231 proliferative activity ( Fig. 2e ). In agreement with the Ki-67 analysis, MDA-MB-231 cell number in μTSA was inhibited by surrounding NHDF cells ( Fig. 2f ). With the combined use of μTSA and transwell cell culture inserts, we designed a series of conditions that dissected individual elements in the NHDF inhibition, and found that both soluble factors and direct heterotypic cell–cell contact contributed to the inhibition ( Supplementary Fig. 2 ). 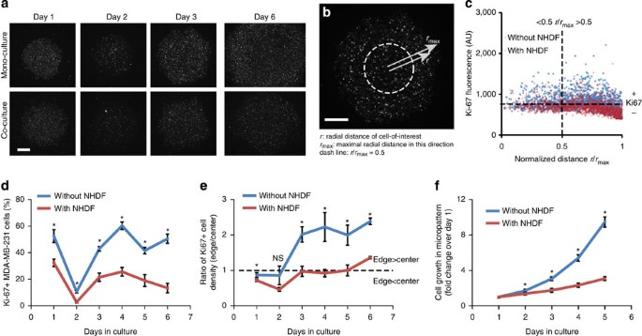Figure 2: Ki-67 expression in MDA-MB-231 cells is spatially regulated and inhibited by NHDF cells in micropatterned cultures. (a) Images of Ki-67 staining in MDA monoculture and co-culture with NHDF over 6 days. (b) Image analysis of Ki-67 positivity in μTSA.r: radial distancerof a cancer cell from the centre of micropattern;rmaxcentre-to-edge distance along the same vector direction; dash line:r/rmax=0.5 separates cancer cell region into central and edge areas (see Methods). (c) Cellular Ki-67 staining intensities were plotted against normalized distances, and threshold into positive and negative cells. (d) Percentage of Ki-67+ MDA cells in micropatterns in absence (blue) and presence (red) of surrounding NHDF cells over 6 days. (e) The ratio of the Ki-67+ MDA cell density between micropattern edge (area outside dash line) and centre (area within dash line). (f) MDA cell growth in micropatterns without or with NHDF cells, measured by total GFP intensity in each micropattern area. Scale bar, 500 μm. (d–f) NS, not significant; *P<0.05 by Student’st-test. (d–e)n=3 per condition per day; (f)n=6 per condition. Error bars: s.d. Figure 2: Ki-67 expression in MDA-MB-231 cells is spatially regulated and inhibited by NHDF cells in micropatterned cultures. ( a ) Images of Ki-67 staining in MDA monoculture and co-culture with NHDF over 6 days. ( b ) Image analysis of Ki-67 positivity in μTSA. r : radial distance r of a cancer cell from the centre of micropattern; r max centre-to-edge distance along the same vector direction; dash line: r / r max =0.5 separates cancer cell region into central and edge areas (see Methods). ( c ) Cellular Ki-67 staining intensities were plotted against normalized distances, and threshold into positive and negative cells. ( d ) Percentage of Ki-67+ MDA cells in micropatterns in absence (blue) and presence (red) of surrounding NHDF cells over 6 days. ( e ) The ratio of the Ki-67+ MDA cell density between micropattern edge (area outside dash line) and centre (area within dash line). ( f ) MDA cell growth in micropatterns without or with NHDF cells, measured by total GFP intensity in each micropattern area. Scale bar, 500 μm. ( d – f ) NS, not significant; * P <0.05 by Student’s t -test. ( d – e ) n =3 per condition per day; ( f ) n =6 per condition. Error bars: s.d. Full size image LCM of μTSA uncover spatial phenotypic heterogeneity LCM [20] was uniquely integrated with μTSA to uncover cell-specific behaviour in situ with precise spatial resolution. Cancer cells are proposed to coax the stromal microenvironment into a growth-promoting one by activating resident cells and/or recruiting bone marrow-derived cells [21] , [22] , [23] , which, in turn, promote malignant phenotypes [22] . MCF-7, an oestrogen receptor-positive breast cancer cell line, can metastasize to the bone marrow where bone marrow-derived mesenchymal stromal cells (BMSCs) reside; BMSCs, conversely, are recruited to primary lesions in MCF-7 xenograft tumour models [17] . μTSA co-culture of MCF-7 and BMSC illuminated a heterotypic interface (100–200 μm in width) highly positive for cytokeratins and vimentin, respectively ( Fig. 3a ). With LCM, we microdissected four regions of cells in μTSA defined by their proximity to the heterotypic interface and cell type ( Fig. 3b ). Micropattern design P2 ( Fig. 1c inset) was selected for LCM studies because it provided optimal spatial resolution for distinguishing bulk and interfacial cells, as well as cell capture/RNA extraction efficiency from these regions ( Fig. 3c,d ). The extracted RNA had an average RNA integrity number (RIN score) of 8.6 (s.d.=0.64) ( Supplementary Fig. 3 ) out of a scale of 10 (intact RNA) to 1 (totally degraded RNA), which was suitable for gene expression analysis. 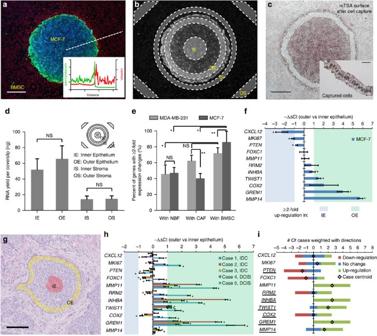Figure 3: Laser capture microdissection (LCM) uncovers spatial phenotypic heterogeneity in μTSA and concordance in human breast cancer tissue. (a) μTSA co-culture of MCF-7 (green: pan-cytokeratin) and bone marrow-derived mesenchymal stromal cell (BMSC; red: vimentin). Nuclei were counterstained with DAPI (4',6-diamidino-2-phenylindole, blue). Inset: line scan of green and red channels from the centre of micropattern into the bulk of BMSC. Scale bar, 500 μm. (b) Four categorical cell regions IE, OE, IS, and OS in μTSA (locations: Inner and Outer; cell components: Epithelium and Stroma) (c) A μTSA co-culture of MCF-7 and BMSC cells after LCM capture of interfacial cancer cells (haematoxylin and eosin). Inset: Captured cells on a thermoplastic membrane. Scale bars, 500 and 100 μm (inset). (d) Average ribonucleic acid (RNA) yield from four regions of a single four-island μTSA co-culture. NS, not significant by Student’st-test. (e) Percent of genes with ≥2-fold expression change in MCF-7 cells out of the 11 genes examined when co-cultured with normal breast fibroblast, cancer-associated fibroblast and BMSC in μTSA. NS, not significant; *P<0.05, by one-way analysis of variance; **P<0.05, by Student’st-test. (f) Relative gene expression change in interface versus bulk in cancer cells. (g) Clinical specimen of human breast cancer (a case of invasive ductal carcinoma (IDC)) and bulk (IE) and interfacial (OE) regions used for LCM and gene expression analysis. Scale bar, 100 μm. (h) Relative expression (−ΔΔCt) of the 11 genes in OE versus IE were plotted in the same way asf. (i) Direction-weighted, stacked numbers of cases for each gene with significant (P<0.05) up- or down-regulations, or no change (P≥0.05). Centroids (diamond) indicate overall direction of gene expression by simple case majority in up- and down-regulations. Underlined genes (7 out of 11, or 63.6%) have matched directions (including no change byPvalue) in μTSA. (f,h) *P<0.05 by Student’st-test, samples had significant changes in gene expression; all other conditions: no significance in gene expression change. (d)n=5–6; (e)n=6; (f,h)n=3. (d–f,h) Error bars: s.d. Figure 3: Laser capture microdissection (LCM) uncovers spatial phenotypic heterogeneity in μTSA and concordance in human breast cancer tissue. ( a ) μTSA co-culture of MCF-7 (green: pan-cytokeratin) and bone marrow-derived mesenchymal stromal cell (BMSC; red: vimentin). Nuclei were counterstained with DAPI (4',6-diamidino-2-phenylindole, blue). Inset: line scan of green and red channels from the centre of micropattern into the bulk of BMSC. Scale bar, 500 μm. ( b ) Four categorical cell regions IE, OE, IS, and OS in μTSA (locations: Inner and Outer; cell components: Epithelium and Stroma) ( c ) A μTSA co-culture of MCF-7 and BMSC cells after LCM capture of interfacial cancer cells (haematoxylin and eosin). Inset: Captured cells on a thermoplastic membrane. Scale bars, 500 and 100 μm (inset). ( d ) Average ribonucleic acid (RNA) yield from four regions of a single four-island μTSA co-culture. NS, not significant by Student’s t -test. ( e ) Percent of genes with ≥2-fold expression change in MCF-7 cells out of the 11 genes examined when co-cultured with normal breast fibroblast, cancer-associated fibroblast and BMSC in μTSA. NS, not significant; * P <0.05, by one-way analysis of variance; ** P <0.05, by Student’s t -test. ( f ) Relative gene expression change in interface versus bulk in cancer cells. ( g ) Clinical specimen of human breast cancer (a case of invasive ductal carcinoma (IDC)) and bulk (IE) and interfacial (OE) regions used for LCM and gene expression analysis. Scale bar, 100 μm. ( h ) Relative expression (−ΔΔCt) of the 11 genes in OE versus IE were plotted in the same way as f . ( i ) Direction-weighted, stacked numbers of cases for each gene with significant ( P <0.05) up- or down-regulations, or no change ( P ≥0.05). Centroids (diamond) indicate overall direction of gene expression by simple case majority in up- and down-regulations. Underlined genes (7 out of 11, or 63.6%) have matched directions (including no change by P value) in μTSA. ( f , h ) * P <0.05 by Student’s t -test, samples had significant changes in gene expression; all other conditions: no significance in gene expression change. ( d ) n =5–6; ( e ) n =6; ( f , h ) n =3. ( d – f , h ) Error bars: s.d. Full size image To reveal instigation of tumour–stromal signalling by stromal cells, expression of 11 cancer progression-related genes focusing on breast cancer cell invasion/migration and stroma activation ( Supplementary Table 1 ) was compared in two breast cancer cell lines (MDA-MB-231, MCF-7) co-cultured with three relevant human fibroblastic stromal cells: (1) normal breast fibroblasts [24] , (2) cancer-associated fibroblasts [24] and (3) BMSCs. BMSCs triggered the most frequent alteration of interfacial gene expression by both tumour cell lines ( Fig. 3e ), supporting a relatively stronger instigation of malignant phenotype by BMSCs. Comparative gene profiling between cells located at the interface versus bulk areas in μTSA showed major differences in BMSC co-culture, where MCF-7 cells had a definitive, spatially resolved gene expression pattern reflecting known in vivo observations ( Fig. 3f ). For example, MMP14 (ref. 25 ), a metalloproteinase used for tumour cell invasion, and TWIST1 (refs 4 , 26 ), an EMT marker indicative of migratory capability, were expressed higher by MCF-7 cells near a BMSC interface compared with bulk, suggesting promotion of cancer cell migration by BMSC through direct-contact or short-range diffusible mediators. These data highlight the ability of a heterotypic tumour–stromal interface to induce localized phenotypic changes that promote malignant progression. Human tumours have concordant phenotypes with μTSA LCM and spatial gene expression analysis were conducted on the 11-gene panel in five ER+ human breast cancer cases, to test whether the localized phenotypic differences relative to the tumour–stromal interface in epithelial compartment observed in the μTSA mimic human patient conditions in vivo . Gene expression of epithelial cells adjacent to a tumour–stroma boundary (outer epithelium, OE) was compared against those near the centre (inner epithelium, IE) in tumour nests with distinct morphological boundaries ( Fig. 3g ). A spatially regulated gene expression pattern emerged as a predominant feature in the epithelium of in vivo tumours ( Fig. 3h ). There was strong concordance with trends of gene expression observed in μTSA compared with the same genes measured in patient cases ( Fig. 3i , 7 underlined genes out of 11 total or 63.6%). A closer look at the magnitude of individual gene changes showed that INHBA , TWIST1 and GREM1 were frequently up-regulated by ≥2-fold (60, 80 and 100% of the cases) in OE in the human tumours ( Fig. 3h ), which were all faithfully recapitulated by μTSA ( Fig. 3f ). Spatially resolved drug action is observed in μTSA The μTSA/LCM system was further evolved to detect unknown, spatially resolved mechanism of action by known cancer therapeutics to disrupt tumour–stromal interactions. In μTSA, we focused on disruption of progression-related tumour–stroma expression profile as an alternative to other forms of cancer drug efficacy (for example, cytotoxicity). Using MCF-7 and BMSC mono-cultures, we pre-screened drugs known to: (1) target bone metastasis (zoledronate, pamidronate) [27] , (2) interrupt stroma-induced tumour growth (reversine [8] ) or (3) modulate BMSC signalling (bortezomib [28] , indomethacin [29] , aspirin [29] , diphenhydramine [30] , rosiglitazone [31] , resveratrol [32] ). The top six drugs were selected according to their ability to maximally disrupt cancer signalling pathways in both cell types ( Supplementary Table 2 ). μTSA of MCF-7 and BMSC were separately treated with the selected drugs ( N =6 μTSAs per drug). LCM-captured cells were analysed for gene expression and compared with the corresponding regions of μTSA without drug treatment ( Fig. 4a ). An aggregated metric, a μTSA gene expression score (see Methods), was introduced to compare drug effects in selective areas and μTSA as a whole. A negative score reflects a strong correlation to an expected inhibitory effect of a given drug against cancer. 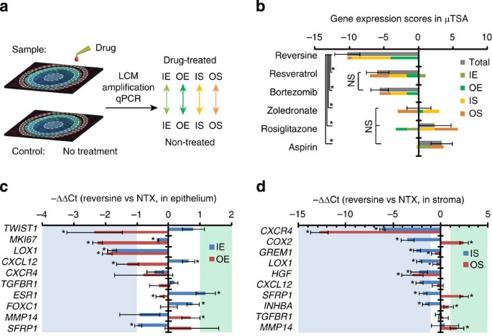Figure 4: Reversine is selected in spatially resolved μTSA drug test with gene expression as readout. (a) Gene expressions in IE, OE, IS and OS were compared between drug treated and non-treated co-cultures of MCF-7 and BMSC in μTSA. (b) A collection of six drugs were tested on the μTSA platform and the scores sorted from negative (cancer-inhibiting) to positive (cancer-promoting), where reversine stood out as the top candidate. Scores from individual regions were plotted in colour bars. NS, not significant between the indicated groups; *P<0.05, by one-way analysis of variance. Gene expression changes in (c) IE and OE and (d) IS and OS caused by reversine treatment. *P<0.05 by Student’st-test, samples had significant changes in gene expression; all other conditions: no significance in gene expression change. (b–d)n=6. Error bars: s.d. Figure 4: Reversine is selected in spatially resolved μTSA drug test with gene expression as readout. ( a ) Gene expressions in IE, OE, IS and OS were compared between drug treated and non-treated co-cultures of MCF-7 and BMSC in μTSA. ( b ) A collection of six drugs were tested on the μTSA platform and the scores sorted from negative (cancer-inhibiting) to positive (cancer-promoting), where reversine stood out as the top candidate. Scores from individual regions were plotted in colour bars. NS, not significant between the indicated groups; * P <0.05, by one-way analysis of variance. Gene expression changes in ( c ) IE and OE and ( d ) IS and OS caused by reversine treatment. * P <0.05 by Student’s t -test, samples had significant changes in gene expression; all other conditions: no significance in gene expression change. ( b – d ) n =6. Error bars: s.d. Full size image Figure 4b depicts μTSA scores arranged in the order of ‘best to worst’ with resolution of regional effects. Reversine stood out as the top candidate; importantly, reversine appeared to primarily affect gene expression at the tumour–stroma interface ( Fig. 4c,d ). Notably, reversine inhibited MCF-7 cell proliferation indicated by Ki-67 expression at the interface but not in the bulk. Though reversine has previously been reported to suppress the growth of multiple myeloma in the presence versus the absence of BMSCs using an in vitro random co-culture [8] , we found in a random co-culture experiment that, while MCF-7 growth was inhibited overall, no additional anti-proliferative effect by reversine was observed in mixed MCF-7/BMSC co-culture compared with MCF-7 monoculture ( Supplementary Fig. 4 ). We further analysed the gene expression change profile in both MCF-7 and BMSC in reversine-treated mixed MCF-7/BMSC co-culture compared with dimethyl sulphoxide (DMSO) treatment by flow sorting ( Supplementary Fig. 5 ). We observed a similar, attenuated profile in response to reversine treatment, as compared with that in the μTSA. In general, mixed co-culture represented an average of μTSA results. These data add to the notion that μTSA can identify drug mechanisms of action that target spatial/interfacial phenomena that are, otherwise, intractable in random co-cultures. In vivo tumour growth is inhibited by reversine We evaluated the activity of reversine on tumour-bearing mice to validate the relevance of μTSA indicated drug mechanisms targeting tumour-stroma interactions in vivo . MCF-7 cells engineered to express firefly luciferase (Luc) were used for in vivo tracking and measurement of organ metastases. We confirmed that luciferase tagging did not alter the MCF-7 phenotype, the response to stromal cells by transwell migration and invasion assays (no transmigration or invasion through membrane with 8 μm pore size, with or without matrigel), or gene expression ( Supplementary Fig. 6 ). MCF-7/Luc cells were injected in the mammary fatpads using matrigel scaffolds in NOD/SCID mice. Tumour-bearing mice were either exposed to reversine or vehicle (DMSO). Tumour growth was monitored over an 8-week period, with an interim analysis at 4 weeks for histological and serological evaluation ( Fig. 5a ). We combined non-invasive and terminal approaches to accurately follow tumour burden. Caliper measurement evaluated the gross physical sizes of the tumours. Terminally extracted tumours at week 4 and 8 were weighed, and biopsies of tumours were homogenized and measured for weight-adjusted luciferase activity ex vivo as a quantification of cancer cell-specific content. Tumour size, measured by caliper, was reduced in the reversine group after 21 days and beyond ( Fig. 5b ; Student’s t -test, P <0.05). Measurement of tumour weights and ex vivo luciferase activity in tumour lysates confirmed that there were increases in tumour size in both treatment groups at week 8, and that a reduction in MCF-7 cancer cell number per tumour by reversine treatment, while insignificant at week 4, became significant at week 8 (Student’s t -test, P =0.002, Fig. 5c ). The primary tumour growth was thus largely unaffected by the reversine treatment until the late stages. 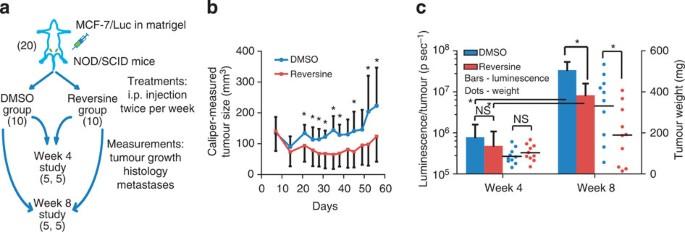Figure 5: Reversine treatment inhibitsin vivotumour growth in a MCF-7 tumour model. (a) MCF-7 cells expressing luciferase were implanted in NOD/SCID mammary fatpads in a total of 20 mice, and monitored for tumour growth with (N=10) and without (N=10) reversine treatment. (b) Tumour growth by caliper measurements. *P<0.05 by Student’st-test; all others: not significant. (c)Ex vivobioluminescent signal and tumour weights measured from extracted tumours at week 4 and 8 (N=5 from each group, respectively). NS, not significant; *P<0.05 by Student’st-test. (b–c) Error bars: s.d. i.p., intraperitoneal. Figure 5: Reversine treatment inhibits in vivo tumour growth in a MCF-7 tumour model. ( a ) MCF-7 cells expressing luciferase were implanted in NOD/SCID mammary fatpads in a total of 20 mice, and monitored for tumour growth with ( N =10) and without ( N =10) reversine treatment. ( b ) Tumour growth by caliper measurements. * P <0.05 by Student’s t -test; all others: not significant. ( c ) Ex vivo bioluminescent signal and tumour weights measured from extracted tumours at week 4 and 8 ( N =5 from each group, respectively). NS, not significant; * P <0.05 by Student’s t -test. ( b – c ) Error bars: s.d. i.p., intraperitoneal. Full size image μTSA predicts reduction of tumour stromalization by reversine We hypothesize that reversine could modify the stromal compartment of tumours on the basis of modulation of tumour–stroma genes observed in μTSA and cause the late tumour growth inhibition. To test this hypothesis, tumour stromalization [33] , defined here as the recruitment of stromal cells and deposition of extracellular matrix components, was quantified by histological metrics. In μTSA tests, LOX1 , which is involved in collagen formation in tumours [34] , was down-regulated in both epithelium and interfacial stroma ( Fig. 3c,d ). Collagen fibres facilitate tumour cell migration, stromal cell infiltration and promote cancer cell growth [35] . In tumour sections rich of cancer cells, the collagen content in the DMSO group was significantly higher and more interspersed than that in the reversine group at week 4 and 8 ( Fig. 6a,b , Student’s t -test, P =0.02 and 0.003). CXCL12 , a cytokine that drives the activation of local fibroblasts [24] and recruited BMSCs [36] into tumour-promoting myofibroblasts [16] , was also found inhibited by reversine at the tumour-stroma interface in μTSA ( Fig. 3c,d ). ELISA analysis of tumour lysates showed a reduction of intratumoral CXCL12 level at week 8 in the reversine group ( Supplementary Fig. 7 , Student’s t -test, P =0.08). Invasion and activation of stromal cells was examined by measuring the density of α-smooth muscle actin (α-SMA) positive cells in tumours. α-SMA is a marker for myofibroblasts, which are promoted by CXCL12 signalling [24] and associated with invasive cancer growth and higher grade malignancy [16] , [37] . The distribution of α-SMA+ cells was largely along the collagen-rich areas ( Fig. 6c ). The percentages of α-SMA+ cells in tumours were different at week 8, but not week 4 ( Fig. 6d ), suggesting a dependence of α-SMA+ cell infiltration on the pre-formation of collagen network. 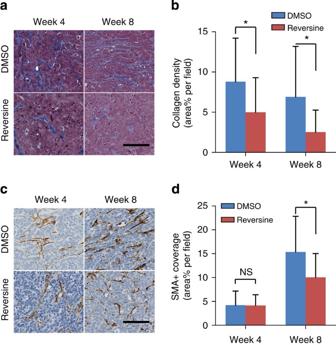Figure 6: Tumour stromalization is reduced by reversine treatment. (a) Masson’s trichrome staining, (b) quantification of collagen density, (c) immunohistochemical α-smooth muscle actin (αSMA) staining and (d) percentage of areas occupied by αSMA+ cells in each field of view. Evaluations were made in tumour areas dominated by cancer cells at week 4 and 8 in the control and reversine treatment groups. Images were taken at 20 × magnification representing five tumours per group. Image numbers analysed (week 4 DMSO, week 4 reversine, week 8 DMSO, week 8 reversine):n=21, 22, 27 and 24 for collagen density;n=35, 55, 129 and 92 for SMA. (a,c) Scale bars, 100 μm. (b,d) Error bars: s.d. NS, not significant; *P<0.05 by Student’st-test. Figure 6: Tumour stromalization is reduced by reversine treatment. ( a ) Masson’s trichrome staining, ( b ) quantification of collagen density, ( c ) immunohistochemical α-smooth muscle actin (αSMA) staining and ( d ) percentage of areas occupied by αSMA+ cells in each field of view. Evaluations were made in tumour areas dominated by cancer cells at week 4 and 8 in the control and reversine treatment groups. Images were taken at 20 × magnification representing five tumours per group. Image numbers analysed (week 4 DMSO, week 4 reversine, week 8 DMSO, week 8 reversine): n =21, 22, 27 and 24 for collagen density; n =35, 55, 129 and 92 for SMA. ( a , c ) Scale bars, 100 μm. ( b , d ) Error bars: s.d. NS, not significant; * P <0.05 by Student’s t -test. Full size image Decrease of metastases by reversine is bone marrow-specific Metastasis, a watershed event in cancer progression [38] , [39] , represents an important end point in the study. Tumour metastatic potential is highlighted by TWIST1 (ref. 40 ) and COX2 (refs 41 , 42 ), which were both down-regulated in μTSA at the interface in epithelial and stromal cells, respectively ( Fig. 3c,d ). We harvested peripheral organs and measured luciferase activity in tissue lysates as an indicator of metastasis. Using a serial dilution of MCF-7/luc cells, we observed high linearity between luciferase activity in lysate versus cell numbers ( Supplementary Fig. 8a ). We determined that this method had a limit of detection (LOD) of three cells per mg tissue sample under our experimental settings, which was used as threshold value to detect the existence of micrometastases in both treatment groups at week 4 and 8. While no discernible metastases were found in week 4 groups, a number of organs were positively detected of cancer cells at the end of an 8-week study in both groups ( Supplementary Fig. 8b , summarized in Table 1 ), confirmed by immunohistochemical (IHC) staining of human mitochondria ( Supplementary Fig. 9 ). Intriguingly, we detected no bone metastasis in any reversine-treated mice compared with 60% of mice in the DMSO group ( Table 1 ). The blockade of bone metastasis was organ-specific, as cancer cells were detected in other organs at a similar frequency when comparing groups. Table 1 Reversine treatment leads to bone marrow-specific reduction of metastases detected at week 8. Full size table The tumour–stromal interface is known to co-evolve with epithelial cancer from pre-invasive to malignant stages [43] . The mechanism of interfacial interactions in driving progression and the implication for cancer therapeutics are, however, largely unknown. To mimic the structurally constrained tumour–stromal interactions in vivo , we established μTSA as an enabling tool to probe tumour–stromal interfacial phenomena. Micropatterning allows for precise positioning of cell components according to their relative location in tumours, with simultaneous control over cell types, the number and ratio of cells, the degree of cell–cell interactions and the accessibility of one cell to interact with another. The physical layout of cell–cell interactions on a two-dimensional (2D) surface integrates seamlessly with high-content microscopy imaging to allow for real-time and long-term monitoring of cell behaviours and signalling events with phenotypic markers and reporters. LCM was used for molecular profiling of cells in regions of interest to detect signalling changes in response to cell–cell interactions and drug interventions. The use of μTSA with other single-cell capture technologies including micromanipulators and optical trapping can also be envisioned for different applications. In a μTSA model of MCF-7/BMSC, there was a boundary layer of the order of 1–10 cells in width with altered phenotypic expressions in cancer and stromal cells compared with the bulk areas ( Fig. 3a ). LCM and gene expression analysis revealed an array of signalling pathways that were differentially regulated at the interface versus the bulk, particularly in the epithelial compartment. Notably, such localized, spatial phenotypic distributions were observed in human oral squamous cell carcinoma [44] , and cervix and colon carcinomas [45] at similar length scales. This underscores the structurally/spatially regulated interfacial signalling as a potential mechanism widely applicable for the malignant transformation of the tumour microenvironments, as well as for the cancer field effect [46] . Future development of μTSA tumour models with various cancer and stromal types, and micropattern designs mimicking their physical parameters at different cancer stages will enable a systems-level revelation of interfacial signalling in a broad range of cancer types and stages. Conversely, an important application of the μTSA model will also be to validate and study the biological functions of oncogenes [47] and clinically discovered biomarkers [3] . Intratumour heterogeneity has important consequences in promoting tumour evolution and causing therapeutic failure [48] . A notable strength of the μTSA is thus in its ability to model the spatial phenotypic heterogeneity, and identify how drugs differentially modulate cells with regard to their location relative to an epithelial–stromal interface. For instance, reversine had markedly inhibitory effects in the interfacial cells compared with the bulk; resveratrol and bortezomib evenly influenced the different spatial regions; rosiglitazone had opposite overall impacts on epithelial and stromal compartments ( Fig. 4b ). Studying drug dose–response and combinatorial effects in μTSA will therefore contribute to the development of more effective therapeutic regimens. These applications demand high-throughput usage of μTSA either in direct functional readout or downstream analyses. The current platform requires serial extraction of cells of interest with LCM equipment that limits operational efficiency and material yields. We were thus only able to analyse a limited number of genes at a time ( Fig. 3e,f ), or rely on amplification, which introduces an additional complicated process before analysis. One adaptation of the platform will be to improve the engineering design of the co-culture substrate that can allow automated cell separation with high spatial accuracy [11] , and the compatibility with current miniaturized assay platforms [49] . Another route is to combine the current μTSA/LCM techniques with high-throughput techniques such as RNA sequencing and gene expression microarrays, as well as systems biology approaches to discover pivotal molecular nodes in the tumour–stromal signalling. The identified targets will then allow the development of a small, but highly relevant array of reporters for drug-screening readouts. Different cancer types may follow distinct biological processes in the disease progression that correspond to different drug sensitivities [50] . The choice of gene targets (as well as stromal cells) thus should conform to the cancer model of interest, and will have significant impact on the drug discovery. In the present μTSA study, we chose a set of genes focusing on breast cancer cell invasion/migration and stroma activation. As a result, reversine was identified as a potential candidate to reduce the stromalization and bone metastasis in the chosen MCF-7/BMSC model. With established clinical reports on a plethora of gene expression signatures from human specimens [51] , [52] , the potential lists include, but are not limited to inflammation [53] , angiogenesis, cell cycle and metabolism [50] . Notably, another key aspect of the gene expression-based drug evaluation in μTSA is the aggregated gene expression score, where the weight scores were non-discriminatory for all the genes in the same category. This was for the consideration of non-linear characteristic of signalling pathways (that is, a specific expression change is not necessarily proportionally reflected in biological outcome) [54] . Until the quantitative contributions of targets are established, such methodology remains practical, and one way to improve the robustness will be to expand the number of independent targets of interest. Reversine is a synthetic purine that was originally discovered capable of dedifferentiating murine myoblasts to regain multipotency [55] . It has recently been found to possess antitumour capabilities, the exact mechanisms of which have not been clearly defined [8] , [56] , [57] , [58] , [59] , [60] , [61] , [62] . The structural analogy of reversine to ATP implies its major function as a kinase inhibitor [8] . In vitro , reversine was found to suppress the expression of cell cycle-related proteins MPS1, Aurora kinase A, B and C, as well as cell growth signalling enzymes JAK2 and SRC [8] , [57] , and induce growth arrest, polyploidy, autophagy and apoptosis [56] , [58] , [60] . In vivo , reversine was shown to mildly inhibit multiple myeloma growth in a mouse model with intravenous injection of tumour cells, but not with subcutaneous inoculation, indicating a role of the native bone marrow stromal environment in reversine-induced anti-myeloma activities [8] . Two more recent studies demonstrated that reversine inhibited subcutaneous human cervical and thyroid cancer cell growth in nude mouse models [61] , [62] . Interestingly, both reports showed a mild, delayed tumour growth inhibition by reversine compared with DMSO treatments, with onsets of inhibition between 19 and 40 days after implantation, similar to the growth dynamics in the current study. However, both studies assumed a cancer cell-directed drug action without further in vivo analyses. The μTSA model suggests a novel drug mechanism by reversine on tumour stromalization and metastasis by targeting tumour–stromal interactions and is supported by our in vivo findings. The current data cannot completely rule out the contribution of direct inhibition of reversine on cancer cells. Future studies will be designed to separate it from the mechanisms targeting tumour–stromal interactions and stromalization. This can be potentially achieved by rescuing the major kinases affected by reversine in tumour cells, which is yet technically challenging due to the multiplicity of reversine targets [59] . It is important to clearly state that μTSA is not designed as an exact re-creation of in vivo tumours and can be improved upon further. In essence, it captures key tumour–stromal interactions in a spatially regulated manner in vitro that mimics the biophysical constraints imposed by tumour morphology in vivo . In our study, we have used μTSA to explore a spatial heterogeneity of gene expression patterns that was validated by comparison with patient tumour tissue samples. Value in the assay was further gained by its application in drug testing and the new perspective on drug action mechanisms with predictive power to in vivo pre-clinical end points. A more comprehensive gene expression study in μTSA with reference to more human cases can strengthen the statistic confidence in our concordance level (~63%) and greatly expand targets that can be explored in μTSA. A further improvement of μTSA to model human cancer will be the extension of this model from 2D to three-dimensional (3D). There have been reports showing that some cell signalling and phenotypes in the in vivo tumour environments only occur in 3D cultures [63] , [64] . In addition, the diffusion of soluble factors, the effect of extended cell shape with associated rearrangements of the cytoskeleton and intercellular connections, and the sensitivity to anticancer drugs can be very different between 2D and 3D environments [65] , [66] . One of the future directions will be to incorporate 3D elements such as matrix embedment and physical constraints on diffusion, while retaining the ability to interface with microscopy-based and/or high-throughput techniques. While doing so, it will be important to observe if genes that were different between μTSA and human tumour samples in vivo (for example, MMP11 ) revert to similar trends or remain discordant before further follow-up. In summary, μTSA uniquely recapitulates the epithelial–stromal invasion front in tumour microenvironments with extensive control over various microenvironmental parameters. μTSA, coupled with LCM, allowed for direct analyses of phenotypic and gene expression changes in a spatially resolved manner. Heterotypic cell–cell interactions were explored across multiple tumour–stroma pairs to optimize the model. We also demonstrated the translational application of μTSA in discovering a new mechanism of chemotherapeutic drugs that target tumour–stromal interactions. A μTSA-selected drug, reversine, was explored for in vivo efficacy and suppressed tumour growth and bone metastasis through reduced stromal activation in agreement with in vitro μTSA test observations. This technology is flexible, scalable and poised to synergize with the ever-growing field of pharmacogenomics as a platform for diagnostic and therapeutic discovery at the tumour–stroma interface. Cells MDA-MB-231 expressing green fluorescent protein (GFP) was a generous gift from Weinberg lab [17] . Normal breast fibroblast and cancer-associated fibroblast were provided by Orimo lab and previously described by Kojima et al. [24] MCF-7 and NHDF were purchased from ATCC. For in vivo studies, MCF-7 cells were engineered to express firefly luciferase with a lentivirus containing luciferase reporter (MCF-7/Luc) following a previous report [67] . Primary human BMSCs were derived from whole human bone marrow aspirates (Lonza) [68] . BMSCs were expanded in alpha-modified Minimum Essential Medium Eagle (alpha-MEM), 20 mg l −1 gentamycin, 10% FBS, 2.5 μg l −1 rhFGF-basic (R&D Systems), 100 U ml −1 penicillin and 100 mg ml −1 streptomycin. All other cells and co-cultures were grown in Dulbecco’s MEM (DMEM) supplemented with 10% FBS, 100 U ml −1 penicillin and 100 μg ml −1 streptomycin. Antibodies Antibodies used for staining included: anti-pan-cytokeratin (clone C11, 1:500) and vimentin (clone D21H3, 1:200) (Cell Signaling), anti-α-smooth muscle actin (α-SMA) (clone 1A4, 1:200) (Dako), anti-Ki-67 (rabbit polyclonal, ab15580, 1:300) (Abcam), anti-CD105-PE (clone SN6, 1:100) (eBioscience), anti-mitochondria (clone 113-1, 1:100) and anti-fibroblast-specific protein-1 (FSP-1; rabbit polyclonal, 07-2274, 1:200) (Millipore). IL-6 ELISA kit was purchased from BD Biosciences. CCL5 DuoSet ELISA kit and mouse CXCL12/SDF-1 alpha Quantikine ELISA Kit were from R&D Systems. Alexa Fluor fluorescent dye-conjugated secondary antibodies were from Life Technologies for immunofluorescent staining. Reagents Aspirin, indomethacin, resveratrol, reversine, rosiglitazone and zoledronic acid were purchased from Sigma-Aldrich. Bortezomib was from LC Laboratories. Pamidronate and diphenhydramine were from Massachusetts General Hospital (MGH) Pharmacy. Duration of drug treatment in vitro was 48 h for all drugs. Concentrations used for drug treatment on the monoculture and co-cultures are based on the half maximal effective concentrations (EC 50 ) of the selected drugs: aspirin: 10 μM (for COX-2 inhibition); bortezomib: 20 nM; diphenhydramine: 10 μM; indomethacin: 40 μM; pamidronate: 20 μM; resveratrol: 20 μM; reversine: 5 μM; rosiglitazone: 100 nM; zoledronic acid: 40 μM. Micropatterned tumour–stromal assay and drug treatment Round glass coverslips (12 mm in diameter, Fisher Scientific) were cleaned by immersion into hot detergent (MP Biomedicals 7X, diluted 1:3 with deionized water), rinsed with deionized water and dried with nitrogen gas. The cleaned coverslips were treated with oxygen plasma (PDC-32G, Harrick Plasma) for 5 min, and silanized for 15 min with 1% N-(2-aminoethyl)-3-aminopropyl-trimethoxy-silane (Sigma) diluted in deionized water immediately before the treatment. The coverslips were then extensively rinsed in deionized water, dried with nitrogen gas, and cured at 100 °C for 1 h. Lab prepared rat tail collagen I [69] was diluted 1 mg ml −1 in 0.1% acetic acid and coated onto glass coverslips overnight, which were then air-dried and sterilized by ultraviolet exposure for 10 min. Stencils were made by cutting circular features of a series of diameters with a laser engraver (Zing Technologies) in a 250 μm-thick silicone sheet (Rogers Corporation). The diameters of circles in P1~P4 were 3, 1.5, 0.75, and 0.375 mm; center-to-center distances were 4, 2, and 1 mm for P2~P4, respectively. The stencils were then thoroughly rinsed in 70% ethanol and deionized water, and air-dried in a sterile environment. Stencils were applied onto coated glass coverslips, and the whole substrate were submerged in 0.2% (w/v) Pluronic F-127 (Sigma) in phosphate-buffered saline (PBS) for 1 h, and rinsed three times in PBS. Substrates were seeded with cancer cells at a density of 1.5 × 10 5 cells cm −2 , incubated for 1 h and rinsed in warm media. After overnight incubation, stencils were removed and the glass coverslips with micropatterned cancer cell areas were rinsed again with warm media and seeded with stromal fibroblastic cells at 2 × 10 4 cells cm −2 , incubated for 30 min and thoroughly rinsed to remove cells landed on the cancer islands. In drug treatment experiments, drugs were applied on μTSA 24 h after the addition of stromal cell and extended for 48 h. Ki-67 positivity analysis in μTSA To quantitatively analyse Ki-67 in the spatial and temporal dimensions, the intensity of Ki-67 staining in individual cells was registered against their locations in the micropattern island (defined as normalized distance of the cells from the centre of the area by the furthest cell in the same direction, r / r max , Fig. 1e ). The positivity was determined by thresholding the intensity against the staining of the surrounding non-proliferative stromal cells, and the whole circular region was divided into two categorical areas—a central area ( r / r max <0.5) and an outer annular area ( r / r max >0.5) representing the proximity to the border. The density of Ki-67 in each area was defined as the total number of Ki-67-positive cells divided by the total cell numbers in that area (determined by nucleus staining). Laser capture microdissection μTSA co-cultures of MCF-7 and MSC samples were rinsed twice with PBS, fixed with 70% ethanol, rinsed with deionized water and stained with haematoxylin and eosin. All aqueous solutions were treated with diethylpyrocarbonate to avoid RNA degradation. The samples were then submerged in xylene and air-dried immediately before being mounted with cell side upon glass slides for microdissection. Cells of interest were captured using a PixCell Iie LCM system (Arcturus Engineering). A cell-capturing cap with a special thermoplastic film was put in contact with μTSA surface and locally melted into cells of interest in vicinity by low energy infrared laser pulses after microscopic visual selection. When the cap was released from the μTSA surface, it brought cells of interest on the film for subsequent RNA extraction processes. RNA extraction and quantitative PCR RNA was extracted with QIAGEN Rneasy Plus Micro kit, and the quality was evaluated by Agilent 2100 Bioanalyzer (Santa Clara, CA). RNA samples were reverse transcribed and amplified with QIAGEN QuantiTect Whole Transcriptome kit into cDNA following manufacturer’s protocol. Real-time quantitative PCRs were conducted with ViiA 7 system (Applied Biosystems). PCR reagents were obtained from QIAGEN. Primers were designed using NCBI Primer-BLAST and synthesized at MGH DNA Core Facility. Primer sequences are as listed in Supplementary Table 3 . LCM and gene expression analysis of clinical specimens Five ER+ breast tumour specimens were obtained from the Massachusetts General Hospital, which were all formalin-fixed paraffin-embedded (FFPE) biopsies. Three of the tissue specimens were classified as invasive ductal carcinoma, and the rest two were ductal carcinoma in situ . LCM were performed in the tumour nest areas with clear morphological boundaries between epithelial and stromal compartments. For each specimen, a total of ten 7-μm tissue sections were microdissected, and RNA was extracted and purified with Arcturus Paradise PLUS FFPE RNA Isolation Kit (Life Technologies) following the manufacturer’s protocol. The purified RNA samples were then reverse transcribed (SuperScript VILO cDNA Synthesis Kit, Life Technologies), pre-amplified (TaqMan PreAmp, Life Technologies), and analysed for the expressions of housekeeping genes and the 11 genes of interest with TaqMan Gene Expression Assays ( Supplementary Table 4 , Life Technologies). The conduct of this work was covered by an approval from the Massachusetts General Hospital Institutional Review Board, and written informed consent was obtained from all the subjects. μTSA gene expression scoring The expression change of each gene (designated as i ) was scored as expression score E i with −1 (down-regulated by ≥2-fold), 0 (between −1 and 1) or 1 (up-regulated by ≥2-fold). On the basis of the biological functions and clinical associations with cancer progression, each gene was also assigned with a weight score W i of −1 (inhibitory or negatively associated with progression), 0 (no or complex association, or redundant with other genes in the list) or 1 (cancer-promoting or positively associated with progression; Supplementary Table 5 ). Multiplying the direction of expression change ( E i ) with its weight ( W i ) indicates the functional impact of a given drug on a specific molecular target, and the sum total score provides an overall evaluation (Σ E i × W i ). Gene expression analysis of random MCF-7 and BMSC coculture To keep cell number/ratio and culture format the same as μTSA, MCF-7 and BMSC were admixed at the ratio of 1:3 and seeded in a 24-well plate at 10,000 MCF-7 and 30,000 BMSC per well. Cells were co-cultured without drugs for 24 h, treated with DMSO or reversine (5 μM) for 48 h, trypsinized, pooled, stained for CD105-PE and sorted for the positive (BMSC) and negative (MCF-7) fractions on a Modified Digital Vantage Cell Sorter at the MGH Flow Cytometry Core Facility. The sorted cells were extracted for RNA with QIAGEN Rneasy Plus Micro kit. RNA was reverse transcribed with SuperScript VILO cDNA Synthesis Kit (Life Technologies), and real-time quantitative PCRs were conducted with ViiA M 7 system (Applied Biosystems) using primer sequences listed in Supplementary Table 3 . Treatment and measurement of MCF-7 xenograft tumour model Six-week old NOD.CB17-Prkdcscid/J female mice were purchased from Jackson Laboratory and maintained in the animal facility at MGH. Experiments were approved by and conducted in accordance with the policies of the Institutional Animal Care and Use Committee of MGH. Mice were implanted subcutaneously behind neck with oestrogen pellets (17β-estradiol, 0.72 mg per pellet, 60-day release, Innovative Research of America). MCF-7 cells expressing luciferase were resuspended in PBS and 1:1 mixed with high-concentration matrigel (BD Bioscience) and injected in the two abdominal mammary fatpads (1 × 10 7 cells per site in 100 μl volume). Twenty animals were evenly assigned into two groups ( n =10 for both DMSO group and reversine group) and subjected to treatments twice a week. Reversine stock solution in DMSO was diluted in saline and injected intraperitoneally in the treatment group at a dose of 0.5 mg kg −1 body weight. Control group was treated intraperitoneally with the same dose of DMSO carrier diluted in saline. Tumours were allowed to growth for 4 to 8 weeks, with half of the population ( n =5 from each group) killed at week 4 and the other half at week 8. Tumour sizes were measured in the following ways: (1) caliper measurement of the two perpendicular (longest/shortest) axes in the x / y plane, with tumour volume calculated as π xy 2 /6 assuming an ellipsoidal shape, (2) ex vivo bioluminescence measurement of luciferase activity per weight of tumour biopsy (1/4 tumours cut along the long and short axes) lysate, and total signal per tumour back-calculated with tumour weights. At weeks 4 and 8, lung, liver, kidney, spleen and hind leg bone from killed animals were snap-frozen in liquid nitrogen for ex vivo luciferase activity assay. Tumours were extracted and cut in halves, with half snap-frozen for luciferase activity assay and the other half fixed in 10% formalin, dehydrated in 70% ethanol and processed for standard immunohistochemical analyses. Detection of metastases by ex vivo luciferase activity assay Tissues of interest were individually pulverized into a fine powder by hand grinding with a dry ice-chilled porcelain mortar and pestle, and transferred to 1.5 ml tubes on dry ice. Ground tissues were weighted and added with Promega Reporter Lysis Buffer, vortexed for 15 min, frozen and thawed three times with alternating liquid nitrogen and 37 °C water bath, and centrifuged at 12,000 g . Twenty microlitres of each supernatant was mixed with 100 μl of Luciferase Assay Reagent (Promega) and measured for luminescence in a non-transparent white plate (Corning) by BioTek Synergy 2 plate reader. The luciferase activity in lysate was shown to have a wide linear range with regard to cell numbers by a twofold dilution series of a known number of MCF-7/Luc cells ( Supplementary Fig. 8a ). The positivity of metastases was determined by LOD calculated with formula [70] : LOD=mean blank +1.635(SD blank )+1.635(SD low concentration sample ), where mean blank and SD blank are the mean and s.d. of the replicates of a blank sample, and SD low concentration sample is the s.d. of the replicates of the sample containing the lowest concentration of the cell lysate. Immunohistochemistry Fixed tumour samples were processed, embedded in paraffin and sectioned in 5 μm thickness by Specialized Histopathology Services at MGH. Tissue sections were stained with haematoxylin and eosin, Masson’s trichrome and antibodies against α-SMA. Images were scanned by Nanozoomer 2.0RS (Hamamatsu, Japan). Collagen density was calculated as the proportion of blue collagen staining in each field of view in the Masson’s trichrome staining. α-SMA density was evaluated similarly by the percentage area covered by α-SMA positive cells in each field of view. Statistical analysis All data are presented in mean±s.d., as stated in the figure legends. Statistical significance was assessed using Student’s t -test for pair-wise comparison and gene expression, χ 2 test for non-parametric comparison and one-way analysis of variance for comparison between multiple (≥3) conditions; P <0.05 was considered as significant. How to cite this article: Shen, K. et al. Resolving cancer–stroma interfacial signalling and interventions with micropatterned tumour–stromal assays. Nat. Commun. 5:5662 doi: 10.1038/ncomms6662 (2014).